Metabolic engineering ofCorynebacterium glutamicumforL-arginine production L -Arginine is an important amino acid for diverse industrial and health product applications. Here we report the development of metabolically engineered Corynebacterium glutamicum ATCC 21831 for the production of L -arginine. Random mutagenesis is first performed to increase the tolerance of C. glutamicum to L -arginine analogues, followed by systems metabolic engineering for further strain improvement, involving removal of regulatory repressors of arginine operon, optimization of NADPH level, disruption of L -glutamate exporter to increase L -arginine precursor and flux optimization of rate-limiting L -arginine biosynthetic reactions. Fed-batch fermentation of the final strain in 5 l and large-scale 1,500 l bioreactors allows production of 92.5 and 81.2 g l −1 of L -arginine with the yields of 0.40 and 0.35 g L -arginine per gram carbon source (glucose plus sucrose), respectively. The systems metabolic engineering strategy described here will be useful for engineering Corynebacteria strains for the industrial production of L -arginine and related products. L -arginine is an industrially important, semi-essential amino acid, which has numerous applications in food and supplementary health food, pharmaceutical and cosmetics industries [1] , [2] . As with other amino acids and valuable chemicals [3] , [4] , [5] , Corynebacterium glutamicum has advantages as an L -arginine producer because it carries strong flux towards L -glutamate formation [6] , [7] . In contrast to Escherichia coli , C. glutamicum does not have the argA and argE genes, but instead possesses the argJ gene encoding N -acetyltransferase, catalyzing two different biochemical reactions in the L -arginine biosynthetic pathway ( Fig. 1 ). Importantly, C. glutamicum lacks L -arginine degrading enzyme, L -arginine deaminase (arginase) found in E. coli , and thus intracellularly produced L -arginine is not actively degraded. Also, the range of carbon sources utilizable by C. glutamicum is relatively broad, and includes both hexoses and pentoses [8] , [9] , [10] . For the overproduction of L -arginine, the repression of the L -arginine biosynthesis operon ( arg ) by the regulator (encoded by argR ) and the feedback inhibition of the N -acetylglutamate kinase (encoded by argB ) by L -arginine were previously removed in C. glutamicum ATCC 13032 (refs 11 , 12 ). Also, genes constituting the arg operon were amplified, increasing the production of L -arginine [11] , [12] . 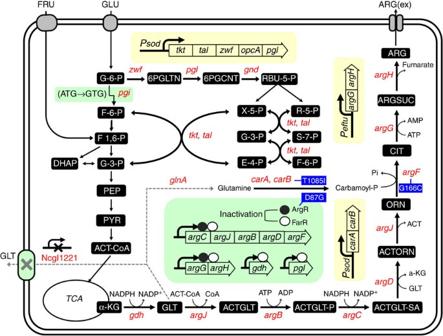Figure 1: Major metabolic pathways associated withL-arginine biosynthesis inC. glutamicumand metabolic engineering approaches applied to overproduceL-arginine. Genes that are knocked out and amplified are shown in green and yellow boxes, respectively, next to their corresponding reactions. The downregulation of thepgigene expression by point mutation is also indicated. Black thick arrows indicate increased fluxes by directly overexpressing the corresponding genes or indirectly by knocking out relevant repressor genes. Dotted grey arrows represent conversion of glutamate to glutamine and the blockage of glutamic acid excretion. Mutated genes leading to amino acid exchanges obtained from AR1 genome sequence are indicated as blue boxes. It should be noted that sucrose without decomposition was used as the carbon source in 5 l bioreactors, while decomposed sucrose (glucose and fructose) was used in 1,500 l bioreactors (Supplementary Table 3). In the case of using non-decomposed sucrose in the cultivation using 5 l bioreactors, the following initial reactions were omitted: import of extracellular sucrose into intracellular sucrose-6-phosphate through the phosphotransferase system (PTS); conversion of sucrose-6-phosphate into glucose-6-phosphate and fructose; export of intracellular fructose to the extracellular space; re-import of fructose into fructose-1-phosphate through the PTS; and conversion of fructose-1-phosphate into fructose-1,6-bisphosphate. 6PGLTN, 6-phosphogluconolactone; 6PGCNT, 6-phosphogluconate; ACT-CoA, acetyl-CoA; ACTGLT, acetylglutamate; ACTGLT-P, acetylglutamyl phosphate; ACTGLT-SA, acetylglutamate semialdehyde; ACTORN, acetylornithine; α-KG, α-ketoglutarate; ARG,L-arginine; ARGSUC, arginosuccinate; CIT,L-citrulline; DHAP, dihydroxyacetone phosphate; E-4-P, erythrose-4-phosphate; F1,6-P, fructose-1,6-bisphosphate; F-1-P, fructose-6-phosphate; F-6-P, fructose-6-phosphate; FRU, fructose; G-3-P, glyceraldehyde-3-phosphate; G-6-P, glucose-6-phosphate; GLT,L-glutamate; GLU, glucose; ORN,L-ornithine; PEP, phosphoenoypyruvate; PYR, pyruvate; R-5-P, ribose-5-phosphate; RIBU-5-P, ribulose-5-phosphate; S-7-P, sedoheptulose-7-phosphate; X-5-P, xylulose-5-phosphate. Figure 1: Major metabolic pathways associated with L -arginine biosynthesis in C. glutamicum and metabolic engineering approaches applied to overproduce L -arginine. Genes that are knocked out and amplified are shown in green and yellow boxes, respectively, next to their corresponding reactions. The downregulation of the pgi gene expression by point mutation is also indicated. Black thick arrows indicate increased fluxes by directly overexpressing the corresponding genes or indirectly by knocking out relevant repressor genes. Dotted grey arrows represent conversion of glutamate to glutamine and the blockage of glutamic acid excretion. Mutated genes leading to amino acid exchanges obtained from AR1 genome sequence are indicated as blue boxes. It should be noted that sucrose without decomposition was used as the carbon source in 5 l bioreactors, while decomposed sucrose (glucose and fructose) was used in 1,500 l bioreactors ( Supplementary Table 3 ). 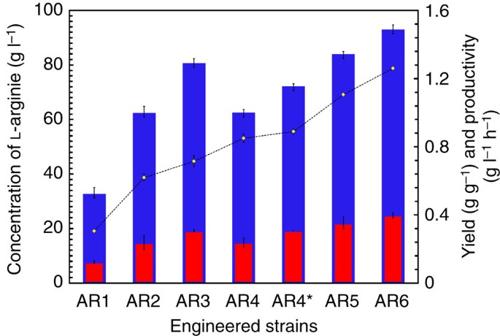Figure 3: Comparison ofL-arginine concentrations, yields and productivities obtained by fed-batch cultivation of engineeredC. glutamicumstrains. Strains AR1, AR2, AR3 and AR4 were cultivated using glucose as a sole carbon source, while AR4 (marked as AR4*), AR5 and AR6 were cultivated using a mixture of glucose and sucrose (1:1 weight ratio) in 5 l bioreactor. The CGAJ medium was used in all these cultivations. Blue and red bars representL-arginine concentration and yield, respectively, while yellow diamond representsL-arginine productivity. Experiments were performed in duplicates. Error bars indicate s.d. In the case of using non-decomposed sucrose in the cultivation using 5 l bioreactors, the following initial reactions were omitted: import of extracellular sucrose into intracellular sucrose-6-phosphate through the phosphotransferase system (PTS); conversion of sucrose-6-phosphate into glucose-6-phosphate and fructose; export of intracellular fructose to the extracellular space; re-import of fructose into fructose-1-phosphate through the PTS; and conversion of fructose-1-phosphate into fructose-1,6-bisphosphate. 6PGLTN, 6-phosphogluconolactone; 6PGCNT, 6-phosphogluconate; ACT-CoA, acetyl-CoA; ACTGLT, acetylglutamate; ACTGLT-P, acetylglutamyl phosphate; ACTGLT-SA, acetylglutamate semialdehyde; ACTORN, acetylornithine; α-KG, α-ketoglutarate; ARG, L -arginine; ARGSUC, arginosuccinate; CIT, L -citrulline; DHAP, dihydroxyacetone phosphate; E-4-P, erythrose-4-phosphate; F1,6-P, fructose-1,6-bisphosphate; F-1-P, fructose-6-phosphate; F-6-P, fructose-6-phosphate; FRU, fructose; G-3-P, glyceraldehyde-3-phosphate; G-6-P, glucose-6-phosphate; GLT, L -glutamate; GLU, glucose; ORN, L -ornithine; PEP, phosphoenoypyruvate; PYR, pyruvate; R-5-P, ribose-5-phosphate; RIBU-5-P, ribulose-5-phosphate; S-7-P, sedoheptulose-7-phosphate; X-5-P, xylulose-5-phosphate. Full size image In this study, we conduct metabolic engineering on the C. glutamicum ATCC 21831 strain that initially undergoes random mutagenesis for the enhanced production of L -arginine [13] . Stepwise rational metabolic engineering based on system-wide analysis of metabolism results in a gradual increase in L -arginine production throughout the strain engineering steps. Fed-batch cultures of our final strain constructed in this study result in the efficient production of L -arginine to the concentrations of 92.5 and 81.2 g l −1 using 5 l and large-scale 1,500 l bioreactors, respectively. Random mutagenesis and inactivation of the repressors C. glutamicum ATCC 21831 strain (AR0 strain hereafter) was chosen as a host strain because of its capability to overproduce L -arginine [13] . When fed-batch culture of the AR0 strain was carried out using glucose as a carbon source, 17 g l −1 of L -arginine was produced ( Supplementary Fig. 1 ). Although the AR0 strain was reported to be already somewhat resistant to an L -arginine analogue, canavanine (CVN) [13] , it was again subjected to random mutagenesis to further increase its tolerance against L -arginine. Cells were treated with N -methyl- N -nitroso- N ′-nitroguanidine and ultraviolet for mutagenesis, and were spread on plates containing increasing concentrations of two L -arginine analogues, arginine hydroxamate (AHX) and CVN, in sequence ( Supplementary Fig. 2 ). Our rationale here is that the production of L -arginine might be further improved by treating greater concentrations of the CVN. Also, although AHX is a frequently used L -arginine analogue in strain development for the enhanced L -arginine production, there has been no record on the use of this analogue to improve the AR0 strain. Thus, it was reasoned that the L -arginine producing capability of the AR0 strain might be further improved (that is, inhibition of negative feedback regulation by L -arginine) by employing both AHX and CVN. Through this random mutagenesis experiment, an AR1 strain resistant to 10 g l −1 of AHX and 30 g l −1 of CVN was isolated ( Supplementary Fig. 3 ). Fed-batch cultivation of the AR1 strain resulted in the production of 34.2 g l −1 of L -arginine, which is more than twofold higher than that obtained with the AR0 strain cultured under the same condition ( Fig. 2a and Supplementary Fig. 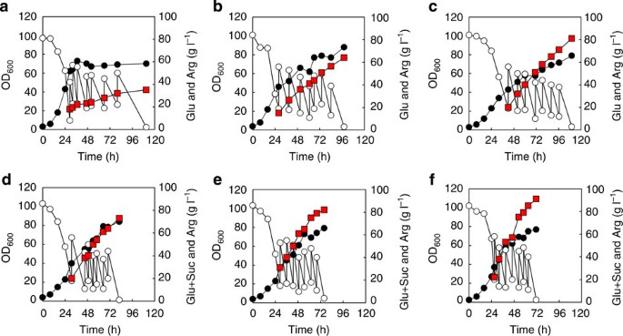4a ). Figure 2: Fed-batch cultures of variousC. glutamicumstrains using bench-scale bioreactors. Shown are the time profiles of cell growth,L-arginine production and carbon source concentration during the fed-batch cultivation of the AR1 (a), AR2 (b) and AR3 (c) strains using glucose as a carbon source, and the AR4 (d), AR5 (e) and AR6 (f) strains using glucose and sucrose (1:1 weight ratio) as dual carbon sources in 5 l lab-scale bioreactor. The CGAJ medium was used in all these cultivations. Closed circle, cell growth (OD600); open circle, glucose (Glu ina–c) and glucose and sucrose (Glu+Suc ind–f); closed red square,L-arginine (Arg). The second set of the fed-batch cultivation data are available inSupplementary Fig. 4. Figure 2: Fed-batch cultures of various C. glutamicum strains using bench-scale bioreactors. Shown are the time profiles of cell growth, L -arginine production and carbon source concentration during the fed-batch cultivation of the AR1 ( a ), AR2 ( b ) and AR3 ( c ) strains using glucose as a carbon source, and the AR4 ( d ), AR5 ( e ) and AR6 ( f ) strains using glucose and sucrose (1:1 weight ratio) as dual carbon sources in 5 l lab-scale bioreactor. The CGAJ medium was used in all these cultivations. Closed circle, cell growth (OD 600 ); open circle, glucose (Glu in a – c ) and glucose and sucrose (Glu+Suc in d – f ); closed red square, L -arginine (Arg). The second set of the fed-batch cultivation data are available in Supplementary Fig. 4 . Full size image To characterize the genetic basis of the AR1 strain exhibiting enhanced L -arginine production capability, the genome sequences of the AR0 and AR1 strains were determined and compared ( Table 1 and Supplementary Data 1–3 ) with our knowledge, the genome sequence of the AR0 strain (that is, ATCC 21831) has not yet been reported. It was found that the AR0 strain possesses a genome distinct from those of other C. glutamicum strains whose whole genome sequences are available ( Supplementary Fig. 5 and Supplementary Data 1 and 2 ). In particular, 293 genes present in the genome of ATCC 13032 strain appeared to be missing in the AR0 strain ( Supplementary Data 1 ) with a large set of potential single-nucleotide polymorphisms (SNPs; Supplementary Data 2 ). With this genomic information of the AR0 strain as a control, pairwise genome alignment for the AR0 and AR1 strains revealed that a total of 580 genes in the AR0 strains appeared to be either deleted or have modified sequences in the AR1 strain ( Supplementary Data 3 ). Among 254 genes annotated with specific functions in the AR0 strain, 18 genes were found to be deleted in the AR1 strain, while remaining 236 genes showed modified sequences in the AR1 strain. Four genes directly related to L -arginine biosynthesis were found to have SNPs in the AR1 strain: argF (ornithine carbamoyltransferase), argJ (bifunctional ornithine acetyltransferase/N-acetylglutamate synthase), argR (arginine repressor) and carB (carbamoyl phosphate synthase large subunit; Fig. 1 ). The argJ gene had a synonymous SNP, having the intact amino acid sequence, while the other genes had nonsynonymous SNPs resulting in a single amino acid change ( Fig. 1 ). Table 1 Comparative genomic analysis of the AR0 and AR1 strains. Full size table The argR and farR genes, both responsible for exerting negative regulation on L -arginine biosynthesis, were inactivated in the AR1 strain to further enhance L -arginine production based on previous report [14] and the comparative genome sequence analysis in the case of the argR gene. ArgR is known to bind to the arg operon ( Fig. 1 ) upon intracellular accumulation of L -arginine beyond its threshold concentration, and inhibits L -arginine biosynthesis [14] , [15] . FarR also represses the expression of the argB , argC , argG , argH , gdh and pgl genes ( Fig. 1 ) in the intracellular presence of L -arginine at high concentration [16] , [17] . Thus, the argR and farR genes were knocked out to construct the AR2 strain, which produced L -arginine to a higher concentration than AR1 by 5 g l −1 in the flask cultivation ( Supplementary Tables 1 and 2 ). Fed-batch culture of the AR2 strain resulted in the production of 61.9 g l −1 of L -arginine ( Fig. 2b and Supplementary Fig. 4b ), which is 28 g l −1 higher than that obtained by the fed-batch culture of the AR1 strain ( Fig. 2a and Supplementary Fig. 4a ). Increasing the NADPH level The NADPH level is one of critical bottlenecks in L -arginine production because the biosynthesis of 1 mol of L -arginine requires 3 mol of NADPH. The adequate intracellular NADPH level is essential in maintaining redox balances in the cell and producing other amino acids required for cell growth [18] . To increase NADPH generation, it was attempted to increase the pentose phosphate pathway (PPP) flux. Thus, the expression level of the pgi gene encoding glucose-6-phosphate isomerase was downregulated by replacing the start codon ATG with GTG, which was reported to reduce its enzyme activity in C. glutamicum [19] , [20] , thereby forcing the metabolic flux towards the PPP; the pgi gene was not knocked out as its complete inactivation results in drastic growth retardation [21] , [22] . Fed-batch culture of the resulting AR3 strain allowed production of 80.2 g l −1 of L -arginine ( Fig. 2c and Supplementary Fig. 4c ), which is 30% greater than that produced by the AR2 strain ( Fig. 2b and Supplementary Fig. 4b ). However, the glucose consumption rate decreased, and consequently the cultivation time was prolonged from 96–111 h. This was thought to be due to the reduced glycolytic flux and non-optimal PPP flux; downregulation of the pgi gene increased metabolic flux entering the PPP, but the flux was not streamlined by the native PPP enzymes. To alleviate this metabolic imbalance causing decreased glucose consumption rate and growth retardation, the PPP genes including the opcA , pgl , tal , tkt and zwf genes ( Fig. 1 ) located in an operon were overexpressed by replacing the native promoter with the strong sod promoter in the AR3 strain to make the AR4 strain. Fed-batch cultivation of the AR4 strain showed that the glucose consumption rate was drastically increased. This resulted in the reduction of fermentation time by 40 h (from 111 to 72 h), and consequently increased L -arginine productivity (0.85 g l −1 h −1 ) compared with those obtained with the AR1 (0.31 g l −1 h −1 ), AR2 (0.62 g l −1 h −1 ) and AR3 (0.72 g l −1 h −1 ) strains ( Fig. 3 ). However, the L -arginine production titre and yield obtained with the AR4 strain were lower than those obtained with the AR3 strain. This was found to be due to the increased biomass formation ( Supplementary Fig. 6 ); thus, cell growth and glucose uptake rates were improved as we intended, but they were improved too much. Figure 3: Comparison of L -arginine concentrations, yields and productivities obtained by fed-batch cultivation of engineered C. glutamicum strains. Strains AR1, AR2, AR3 and AR4 were cultivated using glucose as a sole carbon source, while AR4 (marked as AR4*), AR5 and AR6 were cultivated using a mixture of glucose and sucrose (1:1 weight ratio) in 5 l bioreactor. The CGAJ medium was used in all these cultivations. Blue and red bars represent L -arginine concentration and yield, respectively, while yellow diamond represents L -arginine productivity. Experiments were performed in duplicates. Error bars indicate s.d. Full size image Other than glucose, the most popular carbon source used in industrial fermentation is sucrose (for example, raw sugar from sugar cane). Fed-batch culture of the AR4 strain on sucrose resulted in much reduced cell growth rate (0.41 h −1 ) compared with that (0.75 h −1 ) cultured on glucose. Thus, it was reasoned that the use of a mixture of glucose and sucrose might result in increased production titer and yield of L -arginine by appropriately reducing biomass formation, while maintaining high L -arginine productivity. To test this hypothesis, a mixture of glucose and sucrose (1:1 weight ratio) was employed as a carbon source. Fed-batch culture of the AR4 strain using the mixture of glucose and sucrose resulted in higher production titer (71.7 g l −1 ), yield (0.31 g g −1 ) and productivity (0.89 g l −1 h −1 ) of L -arginine ( Fig. 2d and Supplementary Fig. 4d ) compared with those obtained with glucose as a sole carbon source ( Supplementary Fig. 6 ). Based on these results, a mixture of glucose and sucrose was used in subsequent fermentations. Such simultaneous use of glucose and sucrose has an additional economic advantage in industrial-scale fermentation; the prices of the substrates frequently fluctuate in current market and if two substrates are used, then additional costs incurred from the rise in substrate prices can be mitigated, reducing the economic burden of large-scale fermentation processes. To validate whether the NADPH level was indeed increased as a result of downregulating the pgi gene expression and amplifying the PPP enzymes, the NADPH levels in AR1, AR3 and AR4 strains during their exponential growth phase were measured ( Fig. 4b ). The NADPH level (74.1 μmol gDCW −1 of NADPH) in the AR3 strain, which exhibits downregulated pgi gene expression, was 20% greater than that (54.5 μmol gDCW −1 of NADPH) in the control AR1 strain. The NADPH level in the AR4 strain, in which the PPP genes were overexpressed by using the sod promoter, was even higher at 82.6 μmol gDCW −1 of NADPH. These results confirm that the NADPH level was indeed increased by reinforcing the metabolic flux towards the PPP; downregulation of the pgi gene in the AR3 strain and overexpression of the opcA , pgl , tal , tkt and zwf genes in the AR4 and AR6 (see below) strains increased intracellular concentrations of NADPH compared with the AR1 and AR3 strains ( Fig. 4a ). 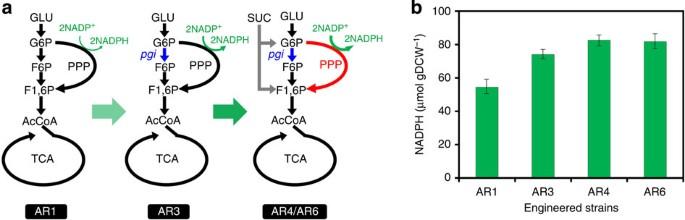Figure 4: Strategies for increasing the NADPH pool. (a) Changes in metabolic fluxes in AR1, AR3, AR4 and AR6 strains. Downregulation of thepgigene (blue arrow) in the AR3 strain and the overexpression of theopcA,pgl,tal,tktandzwfgenes in an operon (red arrow) in the AR4 and AR6 strains led to the increased intracellular NADPH concentration. (b) The NADPH levels in AR1, AR3, AR4 and AR6 strains. The NADPH concentrations were measured from the cells obtained at the exponential growth phases during the 5 l fed-batch fermentation. Experiments were conducted in duplicates. Error bars indicate s.d. Figure 4: Strategies for increasing the NADPH pool. ( a ) Changes in metabolic fluxes in AR1, AR3, AR4 and AR6 strains. Downregulation of the pgi gene (blue arrow) in the AR3 strain and the overexpression of the opcA , pgl , tal , tkt and zwf genes in an operon (red arrow) in the AR4 and AR6 strains led to the increased intracellular NADPH concentration. ( b ) The NADPH levels in AR1, AR3, AR4 and AR6 strains. The NADPH concentrations were measured from the cells obtained at the exponential growth phases during the 5 l fed-batch fermentation. Experiments were conducted in duplicates. Error bars indicate s.d. Full size image Optimization of the L -arginine biosynthetic pathway flux To further optimize L -arginine biosynthetic pathway flux in the AR4 strain, the Ncgl1221 gene, which is known to encode a glutamate exporter in the wild-type C. glutamicum [23] , [24] , was deleted because more L -arginine can be produced if L -glutamate can be converted to L -arginine rather than being excreted into the medium (up to 5 g l −1 ). It should be noted that biotin was included in the medium used in this study ( Supplementary Table 3 ) because C. glutamicum is a biotin auxotroph. Addition of biotin induces this bacterium to produce L -glutamic acid [24] . Flask cultivation of the Ncgl1221-deleted AR4 strain showed similar or slightly better production of L -arginine compared with the AR4 strain ( Supplementary Table 4 ). Next, the sequences of the genes involved in the L -arginine biosynthetic pathway in the AR0, AR1, AR2, AR3 and AR4 strains were examined. The argF gene in AR1 and its derivative strains was found to have a mutation of G166C compared with that in the AR0 strain according to our genome analysis ( Fig. 1 ). This point mutation was obviously introduced during random mutagenesis of the AR0 strain to make the AR1 strain. To examine its effects on cell growth and the L -arginine production capacity, the argF (G166C) was reengineered back to its native gene sequence. The AR4 strain with the native argF gene did not show changes in L -arginine production, but grew faster together with the enhanced carbon uptake rate, which reduced the overall fermentation time by 10 h ( Supplementary Fig. 7 ). This result indicates that the point mutation, argF (G166C), introduced during the random mutagenesis was a negative mutation. Thus, this mutated argF (G166C) was reverted back to its original gene sequence in further strain development. The N-acetylglutamate kinase encoded by the argB gene is known to be feedback inhibited by L -arginine in ATCC 13032 strain, which could be alleviated by two point mutations A26V and M31V [11] . The sequence analysis of the C. glutamicum AR0 strain and its derivatives constructed in this study revealed that the 31st amino acid was already changed to Val. Thus, the 26th amino acid Ala was changed to Val. 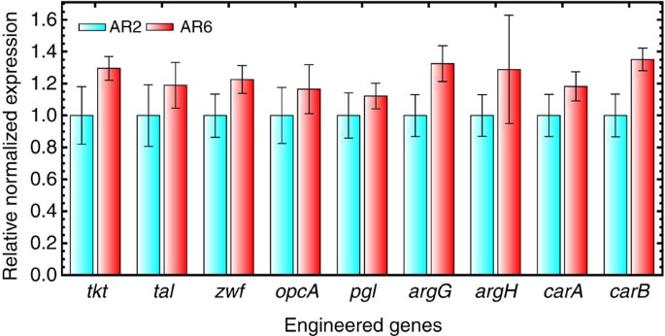Figure 5: Relative normalized expression of the key genes in AR2 and AR6 strains determined by rtPCR. The expression levels of the engineered genes in the AR2 and AR6 strains were determined by rtPCR, and presented as relative normalized expression. The genes examined for their relative expression levels were:tkt, tal, zwf, opcA, pgl, argG, argH, carAandcarB. Experiments were conducted in triplicates, and measurements are represented with their means and s.d. However, this resulted in slower consumption of carbon sources and decrease of L -arginine production ( Supplementary Table 5 ). This result indicates that the argB gene in the AR0 strain is already suitable for L -arginine production without feedback inhibition, differently from the ATCC 13032 strain. 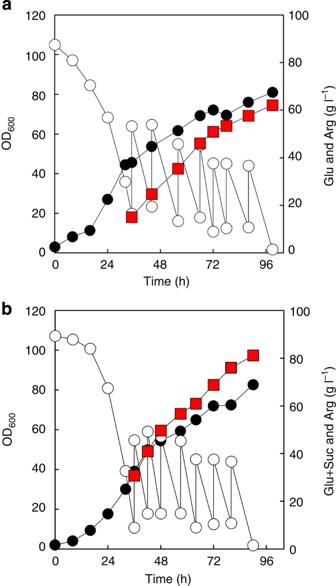Figure 6: Fed-batch cultures ofC. glutamicumAR2 and AR6 strains using pilot-scale bioreactors. Shown are the time profiles of cell growth,L-arginine production and carbon source concentration during the fed-batch cultivation of theC. glutamicumstrains AR2 (a) and AR6 (b) in a 1,500 l large-scale bioreactor. Liquid corn starch was used as a carbon source for cultivating the AR2 strain, while a mixture of liquid corn starch and raw sugar (from sugar cane) at 1:1 ratio (wt) were used for cultivating the AR6 strain. The CGAJ medium was used in all these cultivations. Closed circle, cell growth (OD600); open circle, glucose concentration (Glu ina) and concentration of a mixture of glucose and sucrose (Glu+Suc inb); closed red square,L-arginine concentration (Arg). Next, to increase the availability of carbamoyl phosphate required for converting L -ornithine to L -citrulline by ArgF, the expression levels of the carAB genes were increased by replacing the native promoter with the sod promoter ( Supplementary Table 6 ). It should be noted that the carB gene carried the nonsynonymous SNP in the AR1 strain, compared with the AR0 strain, indicating a potential importance of this gene in enhancing L -arginine production ( Fig. 1 ). Thus, the AR5 strain was constructed by deleting the Ncgl1221 gene, reverting argF (G166C) back to the original sequence, and replacing the native promoter of the carAB genes with the sod promoter in the AR4 strain. Fed-batch culture of the AR5 strain allowed production of 82 g l −1 L -arginine with a yield of 0.35 g g −1 ( Fig. 2e and Supplementary Fig. 4e ), which are greater than those obtained with the AR4 strain ( Fig. 3 ). Debottlenecking the last steps of L -arginine biosynthesis The AR5 strain showed enhanced production of L -arginine, but production of L -citrulline ( ca. 5 g l −1 ), a simultaneously secreted byproduct, persisted. This indicates that the last two enzymes, arginosuccinate synthetase and arginosuccinate lyase, encoded by the argGH genes seem to be rate-controlling. There has been a report showing that the expression levels of the argGH genes were lower than those of the argCJBDF , and even lower in the absence of the argR gene [11] . Since production and excretion of L -citrulline as the byproduct inevitably causes lower L -arginine yield and increased costs for the separation and purification of L -arginine, this problem needs to be solved. Subsequently, the ArgGH flux was increased by replacing the native promoter of the argGH genes with the strong elongation factor Tu (EF-Tu) promoter in the genome of the AR5 strain, resulting in the AR6 strain. It should be noted that C. glutamicum has two biosynthetic gene clusters for L -arginine biosynthesis, argCJBDFR and argGH, under the control of two different promoters ( Fig. 1 ). The NADPH level in the AR6 strain was also found to be 81.8 μmol gDCW −1 , which is comparable to that in the AR4 strain ( Fig. 4b ). Fed-batch culture of the AR6 strain resulted in the production of 92.5 g l −1 L -arginine ( Fig. 2f and Supplementary Fig. 4f ) with a higher yield of 0.40 g g −1 ( Fig. 3 ). L -citrulline was not produced. The concentration, yield and productivity of L -arginine thus achieved are to our knowledge the highest values reported to date. To confirm whether the intended changes in gene expression levels were made in the AR6 strain, microarray analysis of the AR2 (control) and AR6 strains was carried out. The expression levels of the opcA , argG and carAB genes in the AR6 strain were slightly greater than those in the AR2 strain, whereas those of the tkt and tal genes in the AR6 strain were greater by more than twofold and fivefold, respectively, compared with those in the AR2 strain ( Supplementary Table 7 ). To confirm the reduced enzyme activity by downregulating the pgi gene in the AR3-AR6 strains, the PGI activity was measured in the AR6 strain; it was found that the PGI activity in the AR6 strain was decreased by 25%, compared with that in the AR2 strain ( Table 2 ). Because many of these engineered genes showed minor changes in their expression levels, their expression levels in the AR2 and AR6 strains were additionally investigated with real-time PCR (rtPCR). It was confirmed that the expression levels of the engineered genes were modified as intended ( Fig. 5 ). Thus, intended changes in gene expression levels responsible for the observed metabolic alterations could be confirmed by microarray analysis. Table 2 Activities of the PGI in the AR2 and AR6 strains. Full size table Figure 5: Relative normalized expression of the key genes in AR2 and AR6 strains determined by rtPCR. The expression levels of the engineered genes in the AR2 and AR6 strains were determined by rtPCR, and presented as relative normalized expression. The genes examined for their relative expression levels were: tkt, tal, zwf, opcA, pgl, argG, argH, carA and carB . Experiments were conducted in triplicates, and measurements are represented with their means and s.d. Full size image Pilot-scale fermentation of the AR2 and AR6 strains Finally, the large-scale fermentation of the developed AR6 strain was performed, as fermentation performance is known to vary depending on the scale of bioreactors [25] . Fed-batch cultivations of the AR6 and AR2 (control) strains were performed in a 1,500 l bioreactor using corn starch hydrolysate and decomposed raw sugar (containing glucose and fructose; from sugar cane), which are two most popular industrial carbon substrates ( Fig. 6 and Supplementary Fig. 8 ; Supplementary Table 8 ). It should be noted that liquid corn starch hydrolysate was used as a carbon source for cultivating the AR2 strain, while a mixture of liquid corn starch hydrolysate and decomposed raw sugar at 1:1 ratio were used for cultivating the AR6 strain. Different media were used because engineered C. glutamicum strains AR0 to AR3 showed the optimal production performance using glucose as a single carbon source, while the AR4 and subsequent strains showed optimal performance under the medium composed of 50% glucose and 50% decomposed sucrose as carbon sources. Also, it should be noted that sucrose (raw sugar) was decomposed only for this large-scale cultivation because the sucrose uptake of the AR6 strain was slower in the 1,500 l bioreactor than in the 5 l one. Figure 6: Fed-batch cultures of C. glutamicum AR2 and AR6 strains using pilot-scale bioreactors. Shown are the time profiles of cell growth, L -arginine production and carbon source concentration during the fed-batch cultivation of the C. glutamicum strains AR2 ( a ) and AR6 ( b ) in a 1,500 l large-scale bioreactor. Liquid corn starch was used as a carbon source for cultivating the AR2 strain, while a mixture of liquid corn starch and raw sugar (from sugar cane) at 1:1 ratio (wt) were used for cultivating the AR6 strain. The CGAJ medium was used in all these cultivations. Closed circle, cell growth (OD 600 ); open circle, glucose concentration (Glu in a ) and concentration of a mixture of glucose and sucrose (Glu+Suc in b ); closed red square, L -arginine concentration (Arg). Full size image Fed-batch culture of the AR6 strain resulted in 81.2 g l −1 of L -arginine with a yield of 0.353 g g −1 (glucose plus sucrose) and productivity of 0.91 g l −1 h −1 . Thus, the final strain developed by systems metabolic engineering allowed efficient production of L -arginine in large-scale. In comparison, fed-batch culture of the AR2 strain using glucose as a sole carbon source resulted in production of 62.1 g l −1 of L -arginine with a yield of 0.270 g g −1 glucose and productivity of 0.63 g l −1 h −1 . These results suggest that the final AR6 strain, which outperformed the AR2 strain in lab-scale bioreactor, consistently performed much better in a large-scale bioreactor as well. Somewhat lower production performance in 1,500 l fermenter compared with that of the lab-scale fermenter seems to be due to the use of different medium components including industrial grade corn starch hydrolysate, raw sugar and corn steep liquor. L -arginine is an important amino acid that is highly demanded by health, pharmaceutical and industrial markets. Here metabolic engineering of an L -arginine tolerant mutant C. glutamicum strain was performed by systematically knocking out and downregulating the genes that negatively affect L -arginine biosynthesis based on comparative genome analyses, amplifying those that stimulate L -arginine production and optimizing the metabolic fluxes, cofactor availability and the fermentation condition. Although the AR0 strain (that is, ATCC 21831) is known to be an important microbial host for L -arginine production [13] , its genomic and metabolic characteristics have not yet been characterized. Therefore, the genome sequence of the AR0 strain was determined and subjected to comparative genomic analyses. Multiple alignment of genomes of the AR0 strain and seven other C. glutamicum strains revealed that the genome sequence of the AR0 strain is quite different from the other genome sequences ( Supplementary Fig. 5 ). Pairwise alignment between the genomes of the AR0 and ATCC 13032 strains revealed that the AR0 strain does not have at least 293 genes that are present in the ATCC 13032 strain ( Supplementary Data 1 ), the effects of which on the L -arginine production phenotype are not clear. Seven genes involved in the L -arginine biosynthesis of the AR0 strain, including argB , argF , argH , argJ , argR , argS and carA genes, were found to have nonsynonymous SNPs, in comparison with the ATCC 13032 strain, which have likely affected L -arginine production in the AR0 strain ( Supplementary Data 2 ). Relatively large genomic differences between these strains ( Supplementary Fig. 5 ) and mutations in many of these L -arginine biosynthesis-related genes indicate that the AR0 strain seems to be better optimized for the L -arginine overproduction. The genome sequence of the AR1 strain was also determined and compared with that of the AR0 strain, which provided new biological insights and also useful information on potential gene targets to be manipulated. The representative examples include the argR gene knockout, removal of the SNP (that is, G166C) in the argF gene and amplification of the carAB genes. In addition to these genes, the other genes associated with L -arginine biosynthesis in the AR0 strain, having nonsynonymous SNPs compared with those in the ATCC 13032 strain, can be subjected to additional engineering that targets specific base pairs. Genome sequences of the AR0 and AR1 strains deposited in GenBank and their preliminary analysis data provided in this study should serve as a guide for further studies on this strain. From the results of the microarray analyses of the AR2 and AR6 strains, it was not expected to observe that many of the engineered genes appeared to show only minor changes in their expression levels, except for the tkt and tal genes ( Supplementary Table 7 ). These results were also confirmed by additional rtPCR experiments ( Fig. 5 ). It seems that the expression levels of the overexpressed genes might have been affected by their positions in operons [26] , [27] ; genes positioned closer to the promoter were likely to be better expressed than those positioned downstream. The overexpressed genes in an operon involved in the PPP consist of the tkt , tal , zwf , opcA and pgl genes in order, and their expression levels were largely consistent with their relative positions ( Supplementary Table 7 ). This observation was also consistent with the argGH operon, showing that the argG gene was expressed slightly more than the argH gene. The microarray result showing the argR gene expression despite its inactivation (deletion of 99 nucleotides, 21% of the original argR sequence length) seems to be a false positive caused by the hybridization region of the argR gene with its detection probe in the microarray. This probe hybridizes with sequence starting from the first 45 bases of the argR gene, but the in-frame deletion of this argR gene took place from its 131st base. It is notable that the metabolically engineered C. glutamicum developed in this study was capable of efficiently producing L -arginine at large-scale. We want to emphasize the strategies employed for strain and bioprocess development, and in particular, the importance of performing fed-batch culture (which is the preferred industrial standard operation mode) at each critical step during the strain development. This approach not only gave the new targets and objectives for the next round of metabolic engineering, but also prevented the failure of the strain developed at the end without knowing its performance. Most researchers perform flask cultures for evaluating strain performance during the strain development, and perform fed-batch culture for the final strain only. Since strains perform very differently in flask cultures and fed-batch cultures, it is important to examine strain performance in fed-batch culture mode even though the strain is not the final one. This strategy was successfully employed for developing a C. glutamicum strain capable of efficiently producing L -arginine both in lab-scale and large-scale bioreactors. Further studies can be performed for the commercialization of the L -arginine strain. Major considerations include optimizing the culture medium [28] , resolving reduced mass transfer of nutrients in industrial-scale bioreactor [29] and reducing the separation and purification procedure of L -arginine by minimizing byproducts [30] . All these factors substantially affect the overall bioprocess costs, and therefore need to be systematically examined at large-scale, as in the case of pilot-scale cultivation of the AR6 strain conducted in this study. In conclusion, the final C. glutamicum strain developed by systems metabolic engineering was able to efficiently produce L -arginine not only in lab-scale fermentation, but also in large-scale fermentation. Also, genomic studies conducted herein should be useful for the better understanding of this microorganism and further strain development for other applications. Strains and plasmids All bacterial strains, including the genotypes of the constructed AR strains and plasmids used in this study are listed in Supplementary Table 9 . Primers used for the genetic modifications are listed in Supplementary Table 10 . Random mutagenesis and strain isolation Cells were cultured to the OD 600 of 1.0 in a 100 ml flask containing 10 ml CGC medium, washed twice with a saline solution and finally dispersed in 10 ml deionized distilled water (DDW). Then, N -Methyl- N -nitroso- N ′-nitroguanidine was added at 150 μg ml −1 , and cells were incubated at 30 °C and 100 r.p.m. for 10 min. Culture broth after mutagenesis was washed three times with the saline solution, and spread on the plates with CGM medium containing L -arginine analogues, either CVN (10 g l −1 ) or AHX (30 g l −1 ). These plates were incubated for a few days at 30 °C until colonies appeared. Genome analysis of the C. glutamicum strains Genomes of the AR0 and AR1 strains were sequenced using a 454 GS FLX (Roche/454 Life Sciences) at GenoTech Corporation (Daejeon, Korea). A total of 633,303 and 541,313 reads were generated for the AR0 and AR1 strains, respectively, and were assembled into contigs using Newbler ver 2.9. PCR and combinatorial PCR were used to determine the order and direction of the contigs using C. glutamicum ATCC 13032 as a reference strain, and to close the gaps between the contigs. The completed genome sequences had sequence coverages of 82.9 × for the AR0 strain’s chromosome and plasmid and 68.3 × for those of the AR1 strain. The genome sequences were deposited in GenBank ( Table 1 ). Subsequent multiple genome alignment and identification of SNPs were conducted using progressiveMauve [31] and the Artemis Comparison Tool [32] . BLAST ( http://blast.ncbi.nlm.nih.gov/Blast.cgi ) was also conducted to confirm the modified gene sequences in the engineered strains. Fermentation All culture media used in this study are shown in Supplementary Table 3 . Glucose (or corn starch hydrolysate for 1,500 l fermentation) and/or sucrose were used as carbon sources. It should be noted that sucrose was used without decomposition in all lab-scale cultivations using 5 l bioreactors, while decomposed sucrose (raw sugar from sugar cane), which is sucrose decomposed to glucose and fructose through its treatment with phosphoric acid and heat, was used for the cultivation in 1,500 l bioreactor ( Supplementary Table 3 ). In both cases, the relative ratio of glucose and fructose (1:1) was kept the same. All cultivations were performed at 30 °C. Flask cultures for evaluating L -arginine production by different strains were performed as follows. Cells were cultivated on the CGC medium plate for 2 days, and were inoculated into a 100 ml flask containing 10 ml of the 1st seed medium and cultivated in a shaking incubator at 180 r.p.m. for 24 h. One millilitre of the culture was transferred to a 100 ml flask containing 10 ml of the 2nd seed medium and cultured for 24 h. Finally, 1-ml seed culture was transferred into a 100 ml flask containing 10-ml CGAF production medium and cultured for 48 h. Fed-batch cultures were performed in a 5 l bioreactor (Marubishi Corporation) containing 1,800 ml of CGAJ medium at pH 6.8 and 600 r.p.m. The air flow rate was 1 vvm. As described before for the flask cultures, cells cultured on the plate with CGC medium for 2 days were sequentially transferred into 10 ml of the 1st seed medium and then to a 2 l baffled flask containing 200 ml of the 2nd seed medium. This 200 ml seed culture was used to inoculate the bioreactor for fed-batch culture. Additional feed medium was fed into the CGAJ medium when the residual concentration of carbon source became below 20 g l −1 ( Supplementary Table 8 ). Fed-batch cultures were terminated when pH rose, which typically occurred after feeding the feed medium seven times. For the large-scale fed-batch cultivation in a 1,500 l bioreactor, corn starch and sugar cane were used as carbon sources and corn steep liquor as a nitrogen source. Cells cultured in a 70 l bioreactor containing 48 l of the 2nd seed medium were inoculated into a 1,500 l bioreactor containing 600 l of the pilot CGAJ medium. Cells were cultured at the agitation speed of 90 r.p.m., air flow rate of 1 vvm, and pH 6.8. Analytical methods Cell concentration was measured by measuring the absorbance at 600 nm (OD 600 ) using a spectrophotometer (UV-160A; Shimadzu). Residual glucose and sucrose concentrations were measured using a glucose analyzer (YSI 2700 SELECT Biochemistry Analyzer; YSI Life Sciences). The concentration of L -arginine was measured using HPLC (Agilent 1200 series; Agilent Technologies) equipped with a C18 column (Waters) and a fluorescence detector as follows. Samples for the HPLC were prepared by first centrifuging the culture broth and diluting the supernatant to 1:200. A mixture of buffer A and B (7:3) was used as the mobile phase. Buffer A was prepared by dissolving 71.1 g Na 2 HPO 4 ·12H 2 O, 26.8 g CH 3 COONa·3H 2 O and 4 ml acetic acid in 4 l DDW, and adding 260 ml tetrahydrofolate. Buffer B was prepared by mixing methanol, acetonitrile and water at a ratio of 450:100:450, and filtering the mixture. The column temperature was set at 60 °C and the buffer flow rate was 0.4 ml min −1 . Transformation of C. glutamicum AR strains Cells were cultivated in the CGC broth medium overnight, and inoculated into another 50 ml CGC broth at 1% (v/v) and cultivated at 30 °C until the OD 600 of 0.8. Cells were collected by centrifugation at 1,590 g and 4 °C for 10 min, and washed with chilled DDW (at 4 °C). Washed cells were diluted 1:100 with 5 mM HEPES and 15% (v/v) glycerol buffer to set the final culture volume of 500 μl, and aliquoted by 60 μl as competent cells. Cells were transformed with about 2 μg DNA by electroporation (1.8 V and 400 Ω), which was immediately followed by adding 900 μl CGC broth. Cells were incubated for 3 h at 30 °C, and spread on the plates of CGC medium containing 30 mg l −1 kanamycin. Cells were incubated at 30 °C for 3–4 days until colonies appeared. Site-directed mutagenesis Specific modification and engineering of genome, including base substitutions, promoter changes for gene overexpression, and in-frame deletions, were performed as schematically shown in Supplementary Fig. 9 (ref. 33 ). The left and right DNA regions flanking the target gene were individually amplified by PCR, and were combined together by overlapping PCR to create the modified gene fragments. The final construct was cloned into pK19mobsacB containing the sacB gene. When needed, Gibson assembly was used (New England BioLabs). The final gene constructs were selected from the E . coli XL-1-Blue or JM110 as a cloning host. The C. glutamicum AR strains cloned with the above constructed genes were selected with a marker-free system using the Bacillus subtilis sacB gene via two rounds of recombination. The recombinant pK19mobsacB containing the constructed genes was transformed into the AR strains through electroporation, which results in the 1st recombination. The selected colonies were subjected to the 2nd recombination on the plate with CGC medium containing 10% (w/v) sucrose. Modified genotypes in all AR strains ( Supplementary Fig. 9b ) were confirmed by PCR and DNA sequencing. The Ex Taq polymerase (Takara) and the Pfu polymerase (Solgent) were used for amplifying genes by PCR. The restriction and DNA modifying enzymes were purchased from New England BioLabs and used according to the manufacturer’s protocols. DNA ligase was purchased from Takara or Roche. PGI activity assay The C. glutamicum AR2 and AR6 cells cultured in 5 l bioreactor containing the CGAJ medium were harvested at the exponential phase and disrupted by French-Press. The total protein of the cell extract was quantified using the Bradford assay, and the PGI activity level was determined using a colorimetric kit (Cat# MAK103; SIGMA-ALDRICH). The PGI activity was reported in the unit of milliunit ml −1 . One unit of PGI is the amount of enzyme that generates 1.0 μmol of NADH per minute at pH 8.0 at room temperature. NADPH measurement The NADPH levels in the C. glutamicum AR1, AR3, AR4 and AR6 strains were measured using a colorimetric kit (Cat#K347-100; BioVision). Cell extracts were prepared from the exponential growth phase during the fed-batch culture with the CGAJ medium, and intracellular NADPH level was measured by following the absorbance at 450 nm (UV-160A; Shimadzu). Transcriptome analysis Total RNA from C. glutamicum AR2 and AR6 strains, both sampled from the exponential phase of the fed-batch cultivation in the CGAJ medium, was prepared with the RNeasy Mini Kit (Qiagen, Chatworth, CA, USA), and the quality and quantity of RNA were measured by capillary electrophoresis (Agilent Technologies). In the presence of aminoallyl-dUTP and random primers (Invitrogen), complementary DNA (cDNA) probes were prepared by the reverse transcription of the total RNA. The cDNA probes were then purified with Microcon YM-30 column (Millipore) and coupled with Cy5 dye (Amersham Pharmacia). The Cy5-labelled cDNA probes were cleaned up using the QIAquick PCR Purification Kit (Qiagen). Dried Cy5-labelled cDNA probes were resuspended in hybridization buffer. The labelled probes were mixed with RNA on a microarray slide chip ( C. glutamicum ATCC_130323 × 20K; Mycroarray). Hybridization was performed overnight at 42 °C and the slide was washed twice with washing solution 1 (2 × SSC, 0.1%) and washed again with solution 2 (0.1 × SSC, 0.1%). Finally, after chilling at room temperature for 1 min, the slide chip was dried by centrifugation at 400 r.p.m. for 5 min. Hybridization image on the chip was analyzed by GenePix Pro 3.0 software (Axon Instrument). Two independent samples were analyzed, and their measurements were averaged for further analyses. The microarray data were deposited at the Gene Expression Omnibus (GEO) with GEO accession number of GSE52737. rtPCR of the engineered genes The AR2 and AR6 cells were harvested at the exponential phase during the fed-batch cultures. Total RNA was purified using the RNeasy Mini kit (Qiagen, Chatworth, CA). The cDNA was synthesized with Maxime RT PreMix Kit (Cat# 25082; iNtRON). rtPCR was performed using the iQ SYBR Green Supermix (Bio-Rad, Hercules, CA, USA) and the CFX Connect (Bio-Rad). PCR was carried out with 0.5 ng of cDNA template and 10 pM of primers ( Supplementary Table 11 ). The rim and rpoE genes were used as the internal standard. PCR conditions were as follows: 95 °C for 3 min, and subsequent 40 cycles of the three-steps: 95 °C for 30 s, 58 °C for 30 s and 72 °C for 30 s. Accession codes: Gene expression profiles for C. glutamicum strains AR2 and AR6 were deposited in the Gene Expression Omnibus (GEO) under the accession code GSE52737 . Genome sequences of the C. glutamicum ATCC 21831 (or AR0) and AR1 strains were deposited in GenBank/EMBL/DDBJ under the accession codes CP007722 and CP007724 , respectively. How to cite this article: Park, S. H. et al. Metabolic engineering of Corynebacterium glutamicum for L -arginine production. Nat. Commun. 5:4618 doi: 10.1038/ncomms5618 (2014).